Unique behaviour of dinitrogen-bridged dimolybdenum complexes bearing pincer ligand towards catalytic formation of ammonia It is vital to design effective nitrogen fixation systems that operate under mild conditions, and to this end we recently reported an example of the catalytic formation of ammonia using a dinitrogen-bridged dimolybdenum complex bearing a pincer ligand, where up to twenty three equivalents of ammonia were produced based on the catalyst. Here we study the origin of the catalytic behaviour of the dinitrogen-bridged dimolybdenum complex bearing the pincer ligand with density functional theory calculations, based on stoichiometric and catalytic formation of ammonia from molecular dinitrogen under ambient conditions. Comparison of di- and mono-molybdenum systems shows that the dinitrogen-bridged dimolybdenum core structure plays a critical role in the protonation of the coordinated molecular dinitrogen in the catalytic cycle. Nitrogen is an essential element for human beings. To supply the increasing demand of nitrogenous fertilizer, the Haber-Bosch process has long been used industrially to form ammonia from molecular dinitrogen and dihydrogen gasses [1] . The production of ammonia by the Haber-Bosch process requires drastic reaction conditions such as high temperature and high pressure because of the extreme chemical inertness of molecular dinitrogen, although molecular dinitrogen is readily available in plenty from the atmosphere [1] . From a viewpoint of energy, the production of ammonia from molecular dinitrogen and molecular dihydorgen is considered to be the most economical process; however, an enormous amount of energy (over 90% of the total energy of the Haber-Bosch process) was consumed for the production of molecular dihydrogen from fossil fuels. As a result, the development of the alternative to the energy-consuming Haber-Bosch process without the use of molecular dihydrogen has therefore been awaited for a long period of time [1] . Since the discovery of the first example of a transition metal–dinitrogen complex, [Ru(N 2 )(NH 3 ) 5 ] 2+ in 1965 (ref. 2 ), a variety of transition metal–dinitrogen complexes have been prepared, and the reactivity of the coordinated dinitrogen ligand has been studied extensively to exploit a novel catalytic reaction system of molecular dinitrogen by using transition metal–dinitrogen complexes under mild reaction conditions [3] , [4] , [5] , [6] , [7] , [8] , [9] . Among a variety of transition metal–dinitrogen complexes known to date, molybdenum–dinitrogen complexes have intriguing reactivities because the coordinated dinitrogen on the molybdenum atom is easily converted into ammonia by the protonation with inorganic acids such as sulphuric acid, where only a stoichiometric amount of ammonia is produced based on the molybdenum atom [10] , [11] , [12] . In sharp contrast to the stoichiometric transformations, there are only a few examples of catalytic transformations by using transition metal–dinitrogen complexes as catalysts [13] , [14] , [15] , [16] , [17] , [18] , [19] , [20] , [21] . In 2003, Schrock and co-worker found the first example of the catalytic conversion of molecular dinitrogen into ammonia by using molybdenum–dinitrogen complex bearing a triamidoamine as the supporting ligand under ambient conditions, where less than 8 equiv of ammonia were produced based on the molybdenum atom [22] , [23] , [24] , [25] , [26] . Results of the theoretical study on the reaction pathway also support that the catalytic reaction proceeds via some reactive intermediates such as mononuclear hydrazide, -hydrazidium and -nitride complexes [22] , [23] , [24] , [25] , [26] . Quite recently, Peters and co-workers have reported the first successful example of the iron-catalysed direct transformation from molecular dinitrogen into ammonia at −78 °C, where up to 7 equiv of ammonia were produced based on the iron atom of iron–dinitrogen complex bearing a tris(phosphine)borane ligand [27] . Although they have clarified some elementary steps of the catalytic reaction, the whole catalytic cycle has not yet been clarified until now. As an extensive study on the development of novel nitrogen fixation systems under ambient reaction conditions [28] , [29] , [30] , [31] , [32] , [33] , [34] , [35] , [36] , we have recently found another successful example of the catalytic conversion of molecular dinitrogen into ammonia by using dinitrogen-bridged dimolybdenum complex bearing a PNP-type pincer ligand [Mo(N 2 ) 2 ( PNP )] 2 (μ-N 2 ) ( 1 : PNP =2,6-bis(di-tert-butylphosphinomethyl)pyridine), where up to 23 equiv of ammonia were produced based on the catalyst (12 equiv of ammonia based on the molybdenum atom) [37] , [38] , [39] , [40] , [41] . In this paper, we postulate a reaction pathway for the catalytic conversion of molecular dinitrogen into ammonia, where mononuclear molybdenum–dinitrogen complexes bearing the PNP-type pincer ligand have been considered to work as key reactive intermediates. To obtain more detailed information on the reaction pathway, we prepare the mononuclear molybdenum–nitride complexes bearing the PNP-type pincer ligand and examine their catalytic reactivity towards the catalytic formation of ammonia from molecular dinitrogen, because transition metal–nitride complexes are considered to work as key reactive intermediates in the conversion of the coordinated dinitrogen into ammonia [42] , [43] , [44] , [45] , [46] , [47] . We also perform a density functional theory (DFT) study on the reaction pathway based on the stoichiometric and catalytic reactivities of the newly isolated molybdenum complexes bearing the PNP-type pincer ligand. The combined experimental and theoretical studies reveal that the dinitrogen-bridged dimolybdenum core structure plays a crucial role to promote the catalytic reaction in the protonation of the coordinated molecular dinitrogen in the catalytic cycle. This result is in sharp contrast to our previous proposals, where only mononuclear molybdenum complexes were proposed to work as key reactive intermediates [37] , [38] , [39] , [40] , [41] . In this article, we propose a new catalytic reaction pathway with the aid of DFT calculations and experimental results. Preparation and reactivity of molybdenum–nitride complexes As described in the previous paper, we have already prepared a hydrazide complex bearing the PNP-type pincer ligand [Mo(NNH 2 )F( PNP )(C 5 H 5 N)]BF 4 (C 5 H 5 N=pyridine) by the protonation of 1 with tetrafluoroboric acid; however, this hydrazide complex has no catalytic activity towards the catalytic conversion of molecular dinitrogen into ammonia [37] , [38] , [39] , [40] , [41] . As a next step, we paid our attention to the preparation of molybdenum–nitride complexes [42] , [43] , [44] , [45] , [46] , [47] bearing the PNP-type pincer ligand. Treatment of [MoCl 3 (thf) 3 ] with Me 3 SiN 3 at 50 °C for 1 h and then the addition of PNP at 50 °C for 4 h gave a paramagnetic molybdenum(V) nitride complex [Mo(≡N)Cl 2 ( PNP )] ( 2 ) in 43% yield ( Fig. 1a ). A preliminary diffraction study of 2 displays the distorted octahedral molybdenum(V) geometry with the mer - PNP ligand, and the nitride ligand occupied a position trans to one of the chloride ligands (see Supplementary Fig. 1 , Supplementary Tables 1 and 3 and Supplementary Data 1 ). Subsequently, reduction of 2 with 1 equiv of KC 8 in THF at room temperature gave a diamagnetic molybdenum(IV) nitride complex [Mo(≡N)Cl( PNP )] ( 3 ) in 46% yield ( Fig. 1a ). The 1 H NMR of 3 indicates a set of signals for the PNP ligand and its preliminary X-ray study also reveals a distorted square-pyramidal geometry with the PNP and chloride ligands in the basal plane and the nitride ligand in the apical position (see Supplementary Fig. 2 , Supplementary Tables 1 and 4 and Supplementary Data 2 ). The infrared spectrum exhibits a weak ν Mo14N band at 1,031 cm −1 (ν Mo15N =1,003 cm −1 ). To confirm the reactivity of the nitride ligand in 3 , the stoichiometric reaction of 3 with 4 equiv of Cp 2 Co (Cp=η 5 -C 5 H 5 ) and [LutH]OTf (Lut=2,6-lutidine; OTf=OSO 2 CF 3 ) was carried out under Ar atmosphere. As a result, ammonia was produced in 83% yield based on the Mo atom in 3 ( Fig. 1a ). 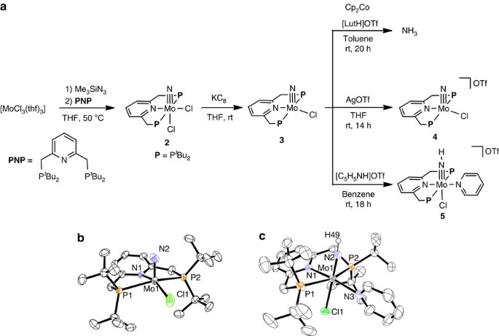Figure 1: Preparation and reactivity of molybdenum–nitride complexes. (a) Preparation and reactivity of2–5. (b) An ORTEP drawing of the cationic part of4. Thermal ellipsoids are shown at the 50% probability level. Hydrogen atoms are omitted for clarity. (c) An ORTEP drawing of the cationic part of5. Thermal ellipsoids are shown at the 50% probability level. Hydrogen atoms except for H49 are omitted for clarity. Figure 1: Preparation and reactivity of molybdenum–nitride complexes. ( a ) Preparation and reactivity of 2 – 5 . ( b ) An ORTEP drawing of the cationic part of 4 . Thermal ellipsoids are shown at the 50% probability level. Hydrogen atoms are omitted for clarity. ( c ) An ORTEP drawing of the cationic part of 5 . Thermal ellipsoids are shown at the 50% probability level. Hydrogen atoms except for H49 are omitted for clarity. Full size image The reaction of 3 with 1 equiv of AgOTf afforded a paramagnetic molybdenum(V) nitride complex [Mo(≡N)Cl( PNP )]OTf ( 4 ) in 52% yield ( Fig. 1a ). The detailed molecular structure of 4 is unambiguously determined by X-ray crystallographic analysis ( Fig. 1b , Supplementary Fig. 3 , Supplementary Tables 2 and 5 and Supplementary Data 3 ). The crystal structure of 4 displays a distorted square-pyramidal geometry, which is closely related to that of 3 . The nitride ligand resides in the apical position, and the Mo≡N bond length is 1.634(3) Å. The chloride ligand is located trans to the nitrogen atom of PNP . Next, the preparation of the molybdenum(IV) imide complex by the protonation of 3 was carried out. Treatment of 3 with 1 equiv of [LutH]OTf in THF gave only unidentified greenish products. When 3 was protonated with 1 equiv of pyridinium trifluoromethanesulphonate [C 5 H 5 NH]OTf as a proton source instead of [LutH]OTf in benzene, a diamagnetic molybdenum(IV) imide complex [Mo(≡NH)Cl( PNP )(C 5 H 5 N)]OTf ( 5 ) was obtained in 53% yield as green crystals ( Fig. 1a ). The 1 H NMR spectrum of 5 exhibits a set of PNP and C 5 H 5 N ligands, while the imide proton could not be assigned. The infrared spectrum of 5 reveals the ν (N−H) band at 3,126 cm −1 . The detailed structure of 5 has been established by an X-ray diffraction study ( Fig. 1c , Supplementary Fig. 4 , Supplementary Tables 2,6 and Supplementary Data 4 ). The molybdenum centre has a distorted octahedral geometry with PNP and C 5 H 5 N in the equatorial plane and mutually trans NH and Cl ligands. The Mo–N (imide) bond length is elongated to 1.711(3) Å from that of 4 . With the nitride and imide complexes bearing the PNP ligand in hand, we have investigated their catalytic activity towards the reduction of molecular dinitrogen into ammonia. When 2 (0.020 mmol) was used as a catalyst in the presence of excess amounts of CoCp 2 (0.72 mmol) and [LutH]OTf (0.96 mmol) under an atmospheric pressure of dinitrogen, only a stoichiometric amount of ammonia was formed based on the molybdenum atom in 2 ( Table 1 , run 2). In contrast, 3 exhibited the catalytic activity to afford 6.6 equiv of ammonia based on the molybdenum atom in 3 , which is comparable to that of 1 ( Table 1 , run 3). Complex 4 also worked as an effective catalyst in contrast to 2 , where 7.1 equiv of ammonia were produced based on the molybdenum atom in 4 ( Table 1 , run 4). On the basis of the results of the stoichiometric and catalytic reactions of newly prepared nitride complexes, we believe that 3 and 4 can be regarded as reactive intermediates in the catalytic reduction of molecular dinitrogen into ammonia. In contrast, no catalytic activity of 2 is considered to be due to the coordination of the second chloro ligand to the molybdenum centre, which may inhibit the generation of the corresponding reactive species. Complex 5 did not work as a catalyst under the same reaction conditions ( Table 1 , run 5). The pyridine ligand coordinated to the Mo atom in 5 is considered to inhibit the generation of reactive species towards the catalytic reaction. In fact, addition of an excess amount (10 equiv) of pyridine to 1 in the catalytic reduction of molecular dinitrogen in the presence of 1 as a catalyst markedly decreased the catalytic activity. This experimental result supports our proposal on the nature of the pyridine ligand in 5 . Table 1 Catalytic formation of ammonia by molybdenum complexes. * Full size table Theoretical calculations We have investigated a possible reaction pathway catalysed by 1 with DFT calculations. On the basis of the above experimental findings, a mononuclear molybdenum(IV) nitride complex [ Mo (≡N)(OTf)] ( Mo =[Mo( PNP )]) can be regarded as a key intermediate. This means that the dinuclear complex [ Mo (N 2 ) 2 ] 2 (μ-N 2 ) 1 must be separated into the corresponding two mononuclear molybdenum complexes at a certain stage in the course of the catalytic reaction. This speculation is reasonable because no dinuclear molybdenum complex except for 1 was experimentally isolated from the catalytic reaction, and the newly prepared mononuclear molybdenum(IV) nitride complex [ Mo (≡N)Cl] 3 was revealed to be capable of serving as a catalyst towards the catalytic formation of ammonia. In our previous report on the transformation of molecular dinitrogen into ammonia catalysed by 1 , we proposed a reaction pathway that 1 is first separated into the corresponding two mononuclear molybdenum–dinitrogen complexes, and then one of the dinitrogen ligands on the Mo atom leads to ammonia [37] . On the basis of computational results obtained in the present paper, we have newly proposed a reaction pathway involving the separation of dinuclear molybdenum complexes after a sequential protonation/reduction of a terminal dinitrogen ligand as well as regeneration of 1 linked with ligand exchange of ammonia for molecular dinitrogen. 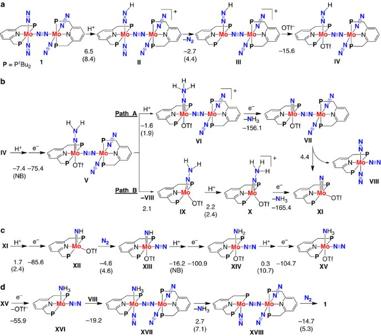Figure 2: A possible reaction pathway by1. (a) Protonation of a terminal dinitrogen ligand in1followed by exchange of the dinitrogen ligandtransto the NNH group for OTf group. Protons and electrons are supplied by lutidinium and cobaltocene, respectively. Energy changes and activation energies (in parenthesis) for individual reaction steps were calculated at the B3LYP*/BS2 level of theory (units in kcal mol−1). NB represents that the corresponding reaction has no activation barrier. (b) A sequential protonation/reduction ofIVand separation of bimetallic complexes leading to formation of ammonia and the monometallic nitride complexXI. (c) A sequential protonation/reduction ofXIvia the six-coordinate imide complexXIIIto give the ammonia complexXV. (d) Ligand exchange of ammonia for molecular dinitrogen leading to regeneration of1. Figure 2 shows a plausible mechanism on the transformation of molecular dinitrogen into ammonia catalysed by 1 via a mononuclear molybdenum–nitride complex as a key intermediate. Detailed information on optimized structures of reactant complexes, transition states and product complexes in individual reaction steps is described in Supplementary Fig. 5 , Supplementary Tables 7–74 and Supplementary Methods . Figure 2: A possible reaction pathway by 1 . ( a ) Protonation of a terminal dinitrogen ligand in 1 followed by exchange of the dinitrogen ligand trans to the NNH group for OTf group. Protons and electrons are supplied by lutidinium and cobaltocene, respectively. Energy changes and activation energies (in parenthesis) for individual reaction steps were calculated at the B3LYP*/BS2 level of theory (units in kcal mol −1 ). NB represents that the corresponding reaction has no activation barrier. ( b ) A sequential protonation/reduction of IV and separation of bimetallic complexes leading to formation of ammonia and the monometallic nitride complex XI . ( c ) A sequential protonation/reduction of XI via the six-coordinate imide complex XIII to give the ammonia complex XV . ( d ) Ligand exchange of ammonia for molecular dinitrogen leading to regeneration of 1 . Full size image Catalytic reaction pathway catalysed by 1 As shown in Fig. 2a , the transformation of molecular dinitrogen into ammonia starts with protonation of a terminal dinitrogen ligand in 1 to form [ Mo (N 2 )(NNH)–N≡N– Mo (N 2 ) 2 ] + II . The dinitrogen ligand trans to the NNH group in II is readily replaced by OTf group that is the counter anion of LutH + ( II → III → IV ). Protonation and one-electron reduction of IV afford a hydrazide(2–) complex [ Mo (OTf)(NNH 2 )–N≡N– Mo (N 2 ) 2 ] V ( Fig. 2b ). After protonation of the hydrazide complex V , reduction of [ Mo (OTf)(NNH 3 )–N≡N– Mo (N 2 ) 2 ] + VI induces a spontaneous N–N bond cleavage to generate the first molecule of ammonia together with [ Mo (OTf)(≡N)–N≡N– Mo (N 2 ) 2 ] VII (Path A in Fig. 2b ). The dinuclear nitride complex VII is readily separated into the corresponding two mononuclear complexes [ Mo (N 2 ) 3 ] VIII and [ Mo (OTf)(≡N)] XI , the latter of which is a key reactive intermediate in the proposed catalytic mechanism (vide infra). When V is separated into the corresponding two mononuclear complexes VIII and [ Mo (OTf)(NNH 2 )] IX , the NNH 2 group in IX is protonated and reduced to afford XI and ammonia ( IX → X → XI ; Path B in Fig. 2b ). Figure 2c describes sequential protonation/reduction steps of XI resulting in the corresponding ammonia complex XV . Protonation/reduction and the coordination of molecular dinitrogen to XI result in the formation of a six-coordinate imide complex [ Mo (OTf)(N 2 )(NH)] XIII ( XI → XII → XIII ). Complex XIII is finally converted into the ammonia complex XV via two sequential protonation/reduction steps ( XIII → XIV → XV ). The proposed catalytic cycle is completed by regeneration of 1 involving exchange of the ammonia ligand for a newly incoming molecular dinitrogen ( Fig. 2d ). Reduction of XV results in a spontaneous elimination of the OTf group. A five-coordinate complex [ Mo (N 2 )(NH 3 )] XVI reacts with complex VIII , generated from dinuclear molybdenum complexes V or VII (vide supra), to afford a dinuclear ammonia complex XVII . Finally, ligand exchange of ammonia in XVII for molecular dinitrogen leads to the regeneration of 1 . Discussion on key steps of the catalytic reaction pathway On the assumption of alternating protonation/reduction steps in the transformation of molecular dinitrogen, one of the dinitrogen ligands in 1 should be protonated at the first step of the catalytic cycle. Since 1 contains four equivalent terminal dinitrogen ligands and one bridging dinitrogen ligand, 1 has at least two reaction sites for the first protonation. Infrared and Raman spectra of 1 indicate that the bridging dinitrogen ligand is more strongly activated and is a better candidate for protonation. However, as shown in Fig. 3a , the protonation of the bridging dinitrogen ligand requires an extremely high activation energy (40.7 kcal mol −1 ), and thus this process does not likely occur at room temperature. In contrast, the activation energy is relatively low (8.4 kcal mol −1 ), although the protonation of a terminal dinitrogen ligand is endothermic by 6.5 kcal mol −1 . A space-filling model of 1 in Fig. 3b indicates that the bridging dinitrogen ligand is sterically protected by eight tert -butyl groups on the phosphorus atoms in the pincer ligands, which make LutH + inaccessible to the bridging dinitrogen ligand without a large distortion around the Mo–N–N–Mo moiety. For the transformation of N 2 into NH 3 catalysed by [HIPTN 3 N]Mo(N 2 ), where HIPTN 3 N=(3,5-(2,4,6-i-Pr 3 C 6 H 2 ) 2 C 6 H 3 N-CH 2 CH 2 ) 3 N, the mechanism of the first protonation/reduction step has been thoroughly investigated [48] , [49] , [50] , [51] . Recent infrared and electron-nuclear double resonance studies reported by Schrock and co-workers [48] , [50] demonstrated that protonation first occurs at an amide nitrogen of the HIPTN 3 N ligand of [HIPTN 3 N]Mo(N 2 ). At present, the most probable reaction pathway for the conversion of [HIPTN 3 N]Mo(N 2 ) into [HIPTN 3 N]Mo(NNH) involves protonation of an amide nitrogen of HIPTN 3 N. The protonated intermediate undergoes reduction and protonation of the N 2 ligand, followed by loss of the first proton from the amide nitrogen. For comparison, we examined protonation of the pyridine nitrogen atom of the pincer ligand. As shown in Fig. 3a , the activation energy for the protonation of the pyridine nitrogen atom is calculated to be 39.1 kcal mol −1 , which is much higher than that of a terminal dinitrogen ligand. In conclusion, the proton transfer from LutH + to 1 should first occur at one of the terminal dinitrogen ligands. 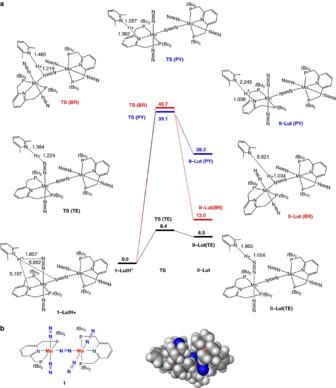Figure 3: The first protonation step of 1. (a) Energy profiles for proton transfer from LutH+to a terminal dinitrogen ligand (TE, black), the bridging dinitrogen ligand (BR, red) and the pyridine nitrogen atom in the pincer ligand (PY, blue) in1. Relative energies are given in kcal mol−1. (b) A space-filling model of1. Figure 3: The first protonation step of 1. ( a ) Energy profiles for proton transfer from LutH + to a terminal dinitrogen ligand ( TE , black), the bridging dinitrogen ligand ( BR , red) and the pyridine nitrogen atom in the pincer ligand ( PY , blue) in 1 . Relative energies are given in kcal mol −1 . ( b ) A space-filling model of 1 . Full size image While the detachment of the proton from the NNH group in II easily occurs ( II → I ; E a =1.9 kcal mol −1 ), the protonation of 1 markedly prompts elimination of the dinitrogen ligand trans to the NNH group. This elimination step is exothermic by 2.7 kcal mol −1 ( E a =4.4 kcal mol −1 ). For comparison, the elimination of an axial dinitrogen ligand in 1 is endothermic by 14.7 kcal mol −1 ( E a =20.0 kcal mol −1 ). After the elimination of the coordinated dinitrogen ligand, OTf group, which is the counter anion of LutH + , will occupy the vacant coordination site of Mo in III to cancel electronic charge of the system ( III +OTf − → IV ; Δ E =–15.6 kcal mol −1 ). This mechanism is feasible since OTf group can exist in the vicinity of III when a terminal dinitrogen ligand in 1 is protonated. The calculated results strongly suggest that the ligand exchange process should be considered as an important part of the first protonation step. Here we should examine the previous proposed reaction pathway [37] , where 1 is first separated into [ Mo (N 2 ) 3 ] VIII and [ Mo (N 2 ) 2 ] XIX , and then a dinitrogen ligand in VIII is protonated towards formation of ammonia (Path C in Fig. 4a ). The bond dissociation energy (BDE) between an Mo centre and the bridging dinitrogen ligand is calculated to be 24.9 kcal mol −1 for 1 , which is much higher than the energy change (+6.5 kcal mol −1 ) for the protonation of a terminal dinitrogen ligand ( Figs 2a and 4a ). Even if the Mo–NN bond dissociation is supposed, the dinitrogen ligands in VIII and XIX do not accept a proton from LutH + . We were not able to obtain any product complex consisting of a protonated VIII and a lutidine molecule, even starting optimization at a H + ˙˙˙N(Lut) distance of 5 Å. Judging from the calculated results, we have newly found that the dinuclear structure remains in the first protonation step. 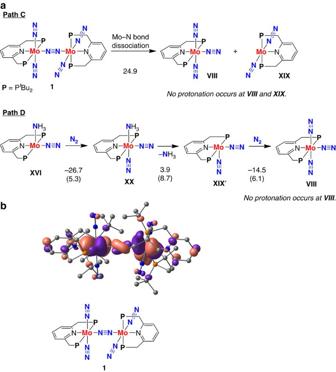Figure 4: An unacceptable reaction pathway by1. (a) An unacceptable reaction pathway on the protonation of the dinitrogen ligands in the mononuclear molybdenum–dinitrogen complexesVIIIandXIX, generated from1, (Path C) and an unsuitable reaction pathway via mononuclear complexes involvingXXas key reactive intermediates (Path D). Energy changes and activation energies (in parenthesis) for individual reaction steps were calculated at the B3LYP*/BS2 level of theory (units in kcal mol−1). (b) Spatial distribution of the HOMO of1. Hydrogen atoms are omitted for clarity. Figure 4: An unacceptable reaction pathway by 1 . ( a ) An unacceptable reaction pathway on the protonation of the dinitrogen ligands in the mononuclear molybdenum–dinitrogen complexes VIII and XIX , generated from 1 , (Path C) and an unsuitable reaction pathway via mononuclear complexes involving XX as key reactive intermediates (Path D). Energy changes and activation energies (in parenthesis) for individual reaction steps were calculated at the B3LYP*/BS2 level of theory (units in kcal mol −1 ). ( b ) Spatial distribution of the HOMO of 1 . Hydrogen atoms are omitted for clarity. Full size image In the proposed catalytic mechanism, formation of [ Mo (OTf)(≡N)] XI is regarded as a key reaction step. To figure out in which steps dinuclear molybdenum complexes are separated, we calculated the BDEs between one Mo centre and the bridging dinitrogen ligand for dinuclear molybdenum complexes 1 , IV , V , VI and VII . As shown in Table 2 , very small BDEs were obtained for the Mo–N α bond of V (2.1 kcal mol −1 ) and VII (4.4 kcal mol −1 ), and therefore these complexes should be separated into the corresponding mononuclear complexes. The small BDEs calculated for V and VII are consistent with the isolation of mononuclear molybdenum hydrazide(2−) complex [ Mo F(NNH 2 )(C 5 H 5 N)]BF 4 (ref. 37 ) and mononuclear molybdenum(IV) nitride complex [ Mo (≡N)Cl] 3 . Table 2 Bond dissociation energies. Full size table Towards the formation of XI , the NNH ligand in IV is first protonated/reduced to give the corresponding hydrazide(2−) complex V . The protonation step is exothermic by 7.4 kcal mol −1 with no activation barrier. We thus exclude a reaction pathway for the protonation of a terminal dinitrogen ligand bound to the other Mo centre in IV . In the reaction pathway via the dinuclear molybdenum–nitride complex VII (Path A in Fig. 2b ), the third protonation to give VI proceeds in an exothermic way with a very low activation barrier (Δ E =−1.6 kcal mol −1 , E a =1.9 kcal mol −1 ). Reduction of VI induces a spontaneous cleavage of the N-NH 3 bond and leads to formation of ammonia together with the dinuclear molybdenum–nitride complex VII . Complex VII undergoes the Mo–N α bond dissociation to give two mononuclear complexes VIII and XI . In the reaction pathway through the mononuclear molybdenum hydrazide(2−) complex IX (Path B in Fig. 2b ), the generated IX is readily protonated ( E a =2.4 kcal mol −1 ) and reduced to afford XI and ammonia. Experimentally, the formation of both dinuclear nitride complex bearing the dinitrogen-bridged dimolybdenum core [ Mo (OTf)(≡N)–N≡N– Mo (N 2 )] and mononuclear nitride complex [ Mo (OTf)(≡N)] was observed by mass spectrometry from the stoichiometric reaction of 1 with 2 equiv of [LutH]OTf in toluene at room temperature. This experimental result supports the proposal of VII and XI by the DFT calculation. The isolated imide complex [ Mo (Cl)(NH)(C 5 H 5 N)]OTf 5 has a six-coordinate structure, in which a pyridine molecule coordinates to the equatorial site of Mo . On the basis of this result, we propose the formation of a six-coordinate imide complex XIII from XI , where the equatorial site of Mo is occupied by an incoming dinitrogen molecule. Because the formation of XIII involves three steps such as protonation, reduction and coordination of molecular dinitrogen, there are three reaction pathways to be considered. One of them is picked up in Fig. 2c . The protonation step leading to XII is found to be slightly endothermic (Δ E =+1.7 kcal mol −1 ), followed by a highly exothermic reduction step. The coordination of molecular dinitrogen to give the six-coordinate XIII also proceeds in an exothermic way (Δ E =−4.6 kcal mol −1 ) with a low activation barrier of 4.6 kcal mol −1 . Other two reaction pathways from XI to XIII are shown in Supplementary Fig. 5 . The imide complex XIII is readily converted to the corresponding amide complex XIV via a barrierless protonation. Further protonation of XIV leading to an ammonia complex XV is almost isoenergetic (Δ E =0.3 kcal mol −1 ) with a moderate activation energy ( E a =10.7 kcal mol −1 ). We discuss the reaction pathway for the exchange of ammonia for molecular dinitrogen in XV involving regeneration of dinuclear complex 1 . As shown in Fig. 2d , reduction of XV induces a spontaneous elimination of the OTf group to give a five-coordinate complex XVI (Δ E =−55.9 kcal mol −1 ). The vacant coordination site in XVI is attacked by [ Mo (N 2 ) 3 ] VIII to form the dinuclear molybdenum ammonia complex XVII . Experimentally, the formation of an ammonia complex bearing the dinitrogen-bridged dimolybdenum core [ Mo (NH 3 )–N≡N– Mo (N 2 ) 2 ] was observed by mass spectrometry from a reaction mixture of the catalytic reaction of 1 with excess amounts of CoCp 2 and [LutH]OTf. This experimental result supports the proposal of XVII by the DFT calculation. Elimination of the coordinated ammonia in XVII yielding [ Mo (N 2 )–N≡N– Mo (N 2 ) 2 ] XVIII is endothermic by only 2.7 kcal mol −1 and requires an activation energy of 7.1 kcal mol −1 . As the final step towards regeneration of 1 , a dinitrogen molecule coordinates to XVIII in an exothermic way (Δ E =−14.7 kcal mol −1 ) with a low activation energy of 5.3 kcal mol −1 . Next, we examined the reaction pathway involving only mononuclear complexes. In this case, as shown in Path D in Fig. 4a , the reaction pathway starts with the coordination of molecular dinitrogen into XVI to give the corresponding mononuclear bis(dinitrogen) complex [ Mo (NH 3 )(N 2 ) 2 ] XX . The dissociation energy of the Mo–NH 3 bond in XX is 3.9 kcal mol −1 . The ligand exchange of ammonia for molecular dinitrogen will be attained in thermal equilibrium; however, the final product complex [ Mo (N 2 ) 3 ] VIII can not be protonated by LutH + (vide supra). Synergy of two molybdenum cores for catalytic ability The calculated results clearly indicate that the mononuclear dinitrogen complex VIII does not serve as an active catalytic species, but that the cooperation between two molybdenum cores in dinuclear complexes plays an essential role in exhibiting the catalytic ability of 1 . In this section, we discuss the reason why the present catalytic system requires the formation of dinuclear complexes in terms of the changes in atomic charge of dinitrogen and their protonated complexes at the first protonation step. Table 3 summarizes differences in atomic charge (Δ q ) between dinitrogen and their protonated complexes obtained for dinuclear ( 1 and II ) and mononuclear ( VIII and XXI ) molybdenum complexes. The atomic charges were calculated with the natural population analysis (NPA) [52] . In the mononuclear system, the NPA charges of the molybdenum centre, the axial dinitrogen ligand, the equatorial dinitrogen ligand and the pincer ligand are increased by 0.38, 0.17, 0.09 and 0.29 after the protonation, respectively. The value of Δ q of NNH (+0.07) is obtained as the charge difference between the NNH group in XXI and the corresponding terminal dinitrogen ligand in VIII . The difference in the total charge is +1 for both systems since one proton is added. Comparison between Δ q ( II – 1 ) of unit A and Δ q ( XXI – VIII ) provides clues as to how unit B in the dinuclear system supports the protonation of the dinitrogen ligand in unit A as a mobile ligand. The values of Δ q calculated for the dinuclear complexes indicate that a large amount of electron (0.34e − ) is donated from unit B to unit A by the protonation. By comparing Δ q ( II – 1 ) of unit A with Δ q ( XXI - VIII ), we are able to figure out that the donated electron mainly distributes on the NNH group (0.10e − ) and the bridging dinitrogen ligand (0.15e − ). The electron transfer between the two molybdenum cores would enhance the Brønsted basicity of the terminal dinitrogen ligand when attacked by LutH + . It is noteworthy that the NPA charges assigned to a terminal dinitrogen ligand in the di- and mononuclear dinitrogen complexes are almost identical (−0.12 for 1 and –0.11 for VIII ). Tanaka et al. [53] previously reported that the NPA charge on a dinitrogen ligand coordinated to a metal atom shows a good correlation with the reactivity of the metal–dinitrogen complex with a proton donor (LutH + ). From a viewpoint of the NPA charge on dinitrogen ligands, the degree of dinitrogen activation of 1 is intrinsically insufficient for the protonation by LutH + . We could not calculate the proton transfer from LutH + to mononuclear dinitrogen complexes such as VIII and XIX . These computational findings suggest that a terminal dinitrogen ligand coordinated to the active molybdenum site in 1 is not ‘preactivated’, but it can receive electron from the other molybdenum core via the bridging dinitrogen ligand only when necessary. Synergy of the molybdenum cores can be understood by looking at the spatial distribution of the HOMO of 1 . As depicted in Fig. 4b , the HOMO of 1 is highly delocalized between d -orbitals of the two molybdenum atoms via a bonding π-orbital of the bridging dinitrogen ligand. The intermetallic electron transfer stemmed from the orbital delocalization allows the dinuclear dinitrogen complex 1 to accept a proton from LutH + at the first step of the catalytic formation of ammonia from molecular dinitrogen. Table 3 Differences in the NPA atomic charge ( Δ q). Full size table Previously we proposed a reaction pathway in which only mononuclear molybdenum–dinitrogen complexes worked as reactive intermediates. On the basis of the present experimental and theoretical studies reported here, we have proposed a new reaction pathway, where the dinuclear structure of the dinitrogen-bridged dimolybdenum–dinitrogen complex plays decisive roles in exhibiting catalytic ability for the transformation of molecular dinitrogen into ammonia. Synergy between the two molybdenum moieties connected with a bridging dinitrogen ligand has been observed at the protonation of the coordinated dinitrogen ligand. A molybdenum core donates electron to the active site of the other core through the bridging dinitrogen ligand, and thereby a terminal dinitrogen at the active site is reductively activated to accept a proton. This means that a mononuclear unit of the dinuclear molybdenum–dinitrogen complex bearing the PNP-type pincer ligands works as a mobile ligand to the other unit as an active site. This result is in sharp contrast to the common role of the dinitrogen-bridged dinuclear metal complexes bearing PNP-type and PCP-type pincer ligands, where dinitrogen-bridged dinuclear metal complexes are known to be used as precursors of mononuclear reactive metal species [54] , [55] , [56] . We consider that our new findings described in this paper provide a new opportunity to design and develop novel and more effective catalytic systems including not only the catalytic formation of ammonia from molecular dinitrogen (nitrogen fixation) but also other catalytic transformations of organic molecules by using dinitrogen-bridged dinuclear metal complexes as catalysts. In addition, we believe that the cooperative activation of molecular dinitrogen by the multinuclear metal complexes described in the present manuscript provides a mechanistic insight to elucidate the reaction pathway in the nitrogenase [3] , [4] , [5] , [6] , [7] , [8] , [9] . General methods 1 H NMR (270 MHz), 31 P{ 1 H} NMR (109 MHz), and 15 N{ 1 H} NMR (27 MHz) spectra were recorded on a JEOL Excalibur 270 spectrometer in suitable solvent, and spectra were referenced to residual solvent ( 1 H) or external standard ( 31 P{ 1 H}: 85% H 3 PO 4 , 15 N{ 1 H}: CH 3 NO 2 ). Infrared spectra were recorded on a JASCO FT/IR 4100 Fourier Transform infrared spectrometer. Absorption spectra were recorded on a Shimadzu MultiSpec-1500. Mass spectra were recorded on a JEOL Accu TOF JMS-T100LP. Elemental analyses were performed at Microanalytical Center of The University of Tokyo. All manipulations were carried out under an atmosphere of nitrogen by using standard Schlenk techniques or glovebox techniques unless otherwise stated. Solvents were dried by the usual methods, then distilled and degassed before use. NaN 2 15 N (Cambridge Isotope Laboratories) was used as received. 2,6-bis(di- tert -butylphosphinomethyl)pyridine ( PNP ) [57] and [MoCl 3 (thf) 3 ] (ref. 58 ) were prepared according to the literature methods. Preparation of [Mo(N)Cl 2 (PNP)] (2) A mixture of [MoCl 3 (thf) 3 ] (125.0 mg, 0.30 mmol) and Me 3 SiN 3 (42 μl, 0.32 mmol) in THF (9 ml) was stirred at 50 °C for 1 h. The resultant dark reddish brown solution was concentrated under reduced pressure. To the residue were added PNP (118.6 mg, 0.30 mmol) and THF (15 ml), and then the mixture was stirred at 50 °C for 4 h. After cooling at room temperature, the orange-brown cloudy solution was passed through glass filter. The solution was cooled at −40 °C to give 2 ·7/3C 4 H 8 O as orange crystals, which were collected by filtration and dried in vacuo to afford 2 (74.5 mg, 0.13 mmol, 43% yield). Anal. Calcd. for C 23 H 43 Cl 2 MoN 2 P 2 : C, 47.92; H, 7.52; N, 4.86. Found: C, 47.35; H, 7.34; N, 4.65. Preparation of [Mo(N)Cl(PNP)] ( 3 ) To a suspension of 2 (57.4 mg, 0.10 mmol) in THF (5 ml) was added KC 8 (13.7 mg, 0.10 mmol), and then the mixture was stirred at room temperature for 20 h. The solution was concentrated under reduced pressure. To the residue was added benzene (3 ml), and the solution was filtered through Celite and the filter cake was washed with benzene (1 ml × 4). The combined filtrate was concentrated to about 3 ml, slow addition of hexane (15 ml) afforded 3 ·1/6C 6 H 14 as dark brown crystals, which were collected by filtration and dried in vacuo to afford 3 (31.5 mg, 0.06 mmol, 58% yield). 31 P{ 1 H} NMR (C 6 D 6 ): δ 98.3 (br s). 1 H NMR (C 6 D 6 ): δ 6.69 (br, ArH, 3H), 3.47–3.41 (m, C H 2 P t Bu 2 , 2H), 3.24–3.18 (m, C H 2 P t Bu 2 , 2H), 1.51 (pseudo t, CH 2 P t Bu 2 , 18H), 1.14 (pseudo t, CH 2 P t Bu 2 , 18H). Infrared (C 6 D 6 , cm −1 ): 1,031 (ν MoN ). Anal. Calcd. for C 23 H 43 ClMoN 2 P 2 : C, 51.07; H, 8.01; N, 5.18. Found: C, 50.72; H, 7.72; N, 5.04. Preparation of [Mo( 15 N)Cl(PNP)] (3- 15 N) A mixture of NaN 2 15 N (49.9 mg, 0.76 mmol) and Me 3 SiCl (190 μl, 1.50 mmol) in THF (3 ml) was stirred at room temperature for 24 h. The resultant white suspension was filtered through Celite and the filter cake was washed with THF (3 ml × 3). To the filtrate was added [MoCl 3 (thf) 3 ] (209.3 mg, 0.50 mmol), and then the mixture was stirred at 50 °C for 1 h. The resultant dark reddish brown solution was concentrated under reduced pressure. To the residue were added PNP (197.4 mg, 0.50 mmol) and THF (20 ml), and then the mixture was stirred at 50 °C for 4 h. After cooling at room temperature, to the reaction mixture was added KC 8 (67.3 mg, 0.50 mmol) and stirred at room temperature for 21 h. The solution was concentrated under reduced pressure. To the residue was added benzene (6 ml), and the solution was filtered through Celite and the filter cake was washed with benzene (2 ml × 4). The combined filtrate was concentrated to ca. 5 ml, and slow addition of hexane (15 ml) afforded 3 - 15 N as dark brown crystals (42.2 mg, 0.08 mmol, 16% yield). 15 N{ 1 H} NMR (THF- d 8 ): δ 737 (s, Mo 15 N ). Infrared (C 6 D 6 , cm −1 ): 1,003 (ν Mo15N ). Preparation of [Mo(N)Cl(PNP)]OTf (4) To a solution of 3 (38.7 mg, 0.072 mmol) in THF (5 ml) was added AgOTf (18.5 mg, 0.072 mmol), and then the mixture was stirred at room temperature for 14 h. The solution was filtered through Celite and the filter cake was washed with THF (2 ml × 3). The combined filtrate was concentrated in vacuo , and the residue was washed with pentane (2 ml × 2). Recrystallization from THF (3 ml)-Et 2 O (20 ml) afforded 4 as yellow crystals (25.5 mg, 0.037 mmol, 52% yield). Calcd. for C 24 H 43 ClF 3 MoN 2 O 3 P 2 S. C, 41.77; H, 6.28; N, 4.06. Found. C, 41.55; H, 6.25; N, 3.97. Preparation of [Mo(NH)Cl(PNP)(C 5 H 5 N)]OTf·C 4 H 8 O (5·C 4 H 8 O) To a solution of 3 (53.8 mg, 0.099 mmol) in C 6 H 6 (5 ml) was added [C 5 H 5 NH]OTf (23.0 mg, 0.100 mmol), and then the mixture was stirred at room temperature for 18 h. The resultant dark green suspension was concentrated in vacuo . The residue was dissolved in THF (3 ml). The solution was filtered through Celite, and the filter cake was washed with THF (1 ml × 3). To the combined filtrate was slowly added Et 2 O (15 ml) to afford 5· C 4 H 8 O as green crystals (44.2 mg, 0.052 mmol, 53% yield). 31 P{ 1 H} NMR (THF- d 8 ): δ 73.9 (s). 1 H NMR (THF- d 8 ): δ 9.58 (d, J =5.1 Hz, 2H), 7.81 (t, J =7.1 Hz, 1H), 7.74–7.64 (m, 3H), 7.40–7.35 (m, 3H), 4.22 (dvt, J =16.2, 4.1Hz, C H 2 P t Bu 2 , 2H), 3.92 (dvt, J =16.2, 4.1Hz, C H 2 P t Bu 2 , 2H), 1.30–1.24 (m, CH 2 P t Bu 2 , 36H). Infrared (KBr, cm −1 ): 3126 (ν NH ). Calcd. for C 33 H 57 ClF 3 MoN 3 O 4 P 2 S. C, 47.06; H, 6.82; N, 4.99. Found. C, 46.76; H, 6.95; N, 4.90. Catalytic reduction of dinitrogen to ammonia under N 2 A typical experimental procedure for the catalytic reduction of dinitrogen into ammonia using the nitride complex 3 is described below. In a 50-ml Schlenk flask were placed 3 (11.0 mg, 0.020 mmol) and 2,6-lutidinium trifluoromethanesulphonate [LutH]OTf (247.1 mg, 0.96 mmol). Toluene (2.5 ml) was added under N 2 (1 atm), and then a solution of CoCp 2 (136.0 mg, 0.72 mmol) in toluene (2.5 ml) was slowly added to the stirred suspension in the Schlenk flask with a syringe pump at a rate of 2.5 ml h −1 . After the addition of CoCp 2 , the mixture was further stirred at room temperature for 19 h. The amount of dihydrogen of the catalytic reaction was determined by GC analysis. The reaction mixture was evaporated under reduced pressure, and the distillate was trapped in dilute H 2 SO 4 solution (0.5 M, 10 ml). Potassium hydroxide aqueous solution (30 wt%; 5 ml) was added to the residue, and the mixture was distilled into another dilute H 2 SO 4 solution (0.5 M, 10 ml). NH 3 present in each of the H 2 SO 4 solutions was determined by the indophenol method [59] . The amount of ammonia was 0.020 mmol of NH 3 collected before base distillation of the reaction mixture and 0.111 mmol of NH 3 collected after base distillation to fully liberate NH 3 , respectively. The total amount of ammonia was 0.131 mmol (6.6 equiv per 3 ). No hydrazine was detected by using the p -(dimethylamino)benzaldehyde method [60] . Reaction of 3 with Cp 2 Co and [LutH]OTf under Ar To a mixture of 3 (21.6 mg, 0.040 mmol), Cp 2 Co (30.3 mg, 0.16 mmol) and [LutH]OTf (41.3 mg, 0.16 mmol) was added toluene (5 ml) under Ar atmosphere, and the mixture was stirred at room temperature for 20 h. The reaction mixture was evaporated under reduced pressure, and the distillate was trapped in dilute H 2 SO 4 solution (0.5 M, 10 ml). Potassium hydroxide aqueous solution (30 wt%; 5 ml) was added to the residue, and the mixture was distilled into dilute H 2 SO 4 solution (0.5 M, 10 ml) under reduced pressure. The amount of NH 3 in each of H 2 SO 4 solution was determined by using the indophenol method. The total amount of NH 3 was 0.033 mmol (0.83 equiv per 3 ). ESI-TOF-MS analysis The reaction of 1 with 2 equiv of [LutH]OTf under N 2 is as follows. To a mixture of 1 (11.0 mg, 0.010 mmol) and [LutH]OTf (5.3 mg, 0.021 mmol) was added toluene (1.5 ml) under N 2 (1 atm), and the mixture was stirred at room temperature for 10 min. The resultant purple suspension was filtered and washed with toluene (1 ml × 2) and dried in vacuo to afford a brownish purple solid. ESI-TOF-MS of the solid in THF showed ion peaks at m/z =1,175.5, which were assigned as those of [Mo(N)(OTf)( PNP )](μ-N 2 )[Mo( PNP )] ( m/z =1,175.4) and at m/z =656.2, which were assigned as those of [Mo(N)(OTf)( PNP )] ( m/z =656.2). During the operation of the isolation of the target complexes, the decomposition of the complexes was observed. The reaction of 1 with excess amounts of Cp 2 Co and [LutH]OTf under N 2 is as follows. To a mixture of 1 (11.3 mg, 0.010 mmol), CoCp 2 (45.8 mg, 0.242 mmol) and [LutH]OTf (82.2 mg, 0.320 mmol) was added toluene (2.0 mL) under N 2 (1 atm), and the mixture was stirred at room temperature for 30 min. The resultant suspension was filtered and the filtrate was concentrated in vacuo to afford a blue solid. ESI-TOF-MS of the solid in THF showed ion peaks at m/z =1,084.5, which were assigned as those of [Mo(NH 3 )( PNP )](μ-N 2 )[Mo(N 2 ) 2 ( PNP )] or [Mo(NH 3 )(N 2 )( PNP )](μ-N 2 )[Mo(N 2 )( PNP )] ( m/z =1,084.4). During the operation of the isolation of the target complex, the decomposition of the complex was observed. Computational methods DFT calculations were performed to search all intermediates and transition structures on potential energy surfaces using the Gaussian 09 program [61] . To estimate the relative energy of different spin states properly, we adopted the B3LYP* functional, which is a reparametrized version of the B3LYP hybrid functional [62] , [63] developed by Reiher and co-workers [64] , [65] . For all intermediates calculated in the present study, the minimum-energy structures have the lowest spin multiplicity (singlet or doublet). The B3LYP and B3LYP* energy expressions are given as equation (1): where a 0 =0.20 (B3LYP) or 0.15 (B3LYP*), a x =0.72, a c =0.81 and in which E X HF is the Hartree-Fock exchange energy; E X LSDA is the local exchange energy from the local spin density approximation; E X B88 is Becke’s gradient correction [66] to the exchange functional; E C LYP is the correlation functional developed by Lee et al. 67 ; and E C VMN is the correlation energy calculated using the local correlation functional of Vosko, Wilk and Nusair (VWN) [68] . For optimization, the LANL2DZ and 6–31G(d) basis sets were chosen for the Mo atom and the other atoms, respectively (BS1). All stationary-point structures were found to have the appropriate number of imaginary frequencies. To determine the energy profile of the proposed catalytic cycle, we performed single-point energy calculations at the optimized geometries using the SDD (Stuttgart/Dresden pseudopotentials) and 6-311+G(d,p) basis sets (BS2). Zero-point energy corrections were applied for energy changes (Δ E ) and activation energies ( E a ) calculated for each reaction step. Solvation effects (toluene) were taken into account by using the polarizable continuum model [69] . All protonation steps by lutidinium (LutH + ) were assessed from a kinetic aspect by exploring reaction pathways. Energy profiles of reduction steps by cobaltocene were calculated based on the following equation, where [XH] + is a protonated intermediate. Accession codes: The X-ray crystallographic coordinates for structures reported in this Article have been deposited at the Cambridge Crystallographic Data Centre (CCDC), under deposition number CCDC 986840, 986841, 973752, 986842. These data can be obtained free of charge from The Cambridge Crystallographic Data Centre via www.ccdc.cam.ac.uk/data_request/cif . How to cite this article: Tanaka, H. et al. Unique behaviour of dinitrogen-bridged dimolybdenum complexes bearing pincer ligand towards catalytic formation of ammonia. Nat. Commun. 5:3737 doi: 10.1038/ncomms4737 (2014).